High-fat maternal diet during pregnancy persistently alters the offspring microbiome in a primate model The intestinal microbiome is a unique ecosystem and an essential mediator of metabolism and obesity in mammals. However, studies investigating the impact of the diet on the establishment of the gut microbiome early in life are generally lacking, and most notably so in primate models. Here we report that a high-fat maternal or postnatal diet, but not obesity per se , structures the offspring’s intestinal microbiome in Macaca fuscata (Japanese macaque). The resultant microbial dysbiosis is only partially corrected by a low-fat, control diet after weaning. Unexpectedly, early exposure to a high-fat diet diminished the abundance of non-pathogenic Campylobacter in the juvenile gut, suggesting a potential role for dietary fat in shaping commensal microbial communities in primates. Our data challenge the concept of an obesity-causing gut microbiome and rather provide evidence for a contribution of the maternal diet in establishing the microbiota, which in turn affects intestinal maintenance of metabolic health. The intestinal microbiome is a robust ecosystem inhabited by nearly 100 trillion bacteria. These commensal bacteria encode enzymatic pathways that enable metabolism and synthesis of fatty acids and vitamins [1] , [2] . It is presumed that at birth vaginal and faecal microbiota from the mother inoculate the oral cavity of the newborn, constituting the foundation of intestinal microbiota in offspring [3] , [4] . As the infant grows and new foods are introduced, the microbiome expands in richness and diversity, reaching a stable state reflective of adult microbiota shortly after weaning [5] , [6] . The influence of maternal gestational diet, mode of delivery and breastfeeding on the phylogenetic structure of the infantile and juvenile intestinal microbiome remains underexplored in well-controlled models [3] , [4] , [5] , [7] . The importance of the establishment and maintenance of host-microbiome symbiosis is underscored by the observation that dysbiotic shifts in microbiota are associated with obesity, inflammatory bowel disorders and an increasing number of autoimmune disorders [1] , [8] , [9] , [10] , [11] , [12] , [13] , [14] , [15] , [16] . Of all environmental factors implicated in structuring the phylogenetic makeup of the microbiome, diet likely plays a predominant role by providing dynamic selective pressure on gut microbes by virtue of substrate availability [17] , [18] , [19] . However, the relative contribution of the host diet and/or habitus on the makeup of the intestinal microbiome remains to be fully elucidated. At the phylum level, Bacteroidetes and Firmicutes compose >90% of the adult intestinal microbiome [2] , [20] . Notably, recent studies indicate that the human gut microbial community is skewed when comparing obese and lean individuals; more specifically, obese individuals tend to harbour a decreased ratio of Bacteroidetes to Firmicutes [1] , [8] , [9] , [15] , [21] , [22] , [23] . Furthermore, when switched to a lean diet, obese individuals lose weight and regain Bacteroidetes [1] , [22] , [23] . In murine models, transplantation of gut microbiota from an obese donor to a germ-free recipient results in a significant increase in body fat percentage after 14 days, which supports a causal role for the intestinal microbiome in increasing host adiposity [1] , [23] . However, these microbiome transplantation experiments were performed between genetically identical mice, and weight gain was only measured over the course of 2 weeks; therefore, these studies may fail to account for genetic heterogeneity thereby masking important gene/diet interactions. More recently, Ridaura et al. [9] colonized germ-free mice with uncultured faecal microbiota or culture collections from human twin pairs discordant for obesity. Interestingly, although microbiota from obese co-twin siblings conferred significantly increased body mass and adiposity when compared with their lean counterpart, there was a significant interaction with the diet of the recipient [9] . Mice fed a diet representative of the upper tertile of saturated fat consumption in the United States, with the lower tertile containing fruits and vegetables, could not be ‘rescued’ by cohousing with a lean colonized littermate [9] . Further, David et al. recently demonstrated how rapidly and drastically the intestinal microbiome can be altered by virtue of diet. The subjects of these studies were provided with both plant-based and animal-based diet for 4 days, and significant alterations in the beta diversity of the microbiome were detected during consumption of the animal-based diet [24] . These alterations in the microbiome correlated to variations in short-chain fatty acids in the faecal content of subjects [24] . These data provided the first line of evidence for strong microbiota-by-diet interactions. In this study, we establish that Mucaca fuscata (Japanese macaque) is a representative model for examining the human microbiome. Further, we are able to examine the role of maternal diet during gestation and lactation in the establishment of the juvenile microbiome. We find that, while the microbiome is structured primarily by virtue of diet, we do find persistent alterations in the juvenile microbiome based on the maternal diet; these persistent alterations occurred despite cohousing of our juvenile cohorts. These studies contribute to the expanding work providing evidence that diet greatly shapes our microbiome. Further, these studies offer insight into how the evolution of the human diet potentially shaped the microbiome to promote incidence of metabolic disease states. Characterization of the Macaca fuscata microbiome To investigate the relative contribution of maternal dietary manipulation and body habitus to the establishment of the microbiome in primates, we undertook metagenomic studies in our well-characterized, outbred Japanese macaque ( Macaca fuscata ) model of maternal obesity [25] , [26] , [27] , [28] , [29] , [30] , [31] , [32] . We first established the comparative relevance of M. fuscata to humans across multiple body sites by collecting oral, vaginal and intestinal samples from healthy, non-gravid adult primates and performing 454 pyrosequencing of 16S rRNA coupled with phylogenetic principal coordinate analysis (PCoA). Akin to the human [2] , [20] , [33] , but unique from the mouse, we observed discrete clustering of oral, vaginal and intestinal microbiota, signifying that these body sites largely harbour unique inhabitant niches, albeit with some individuals demonstrating stool taxa shared within the vagina ( Fig. 1a ). 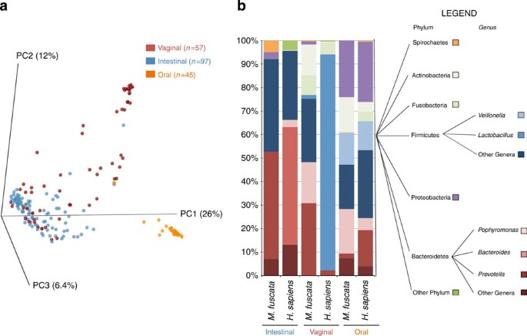Figure 1: Characterization of theMacaca fuscatamicrobiome. DNA was isolated fromM. fuscataorH. sapiensswabs collected from the intestinal (anus, colorectal, and stool), vaginal or oral cavity. 16S rDNA sequencing was performed via the 454 FLXtitanium system and sequences were analysed using QIIME software. (a) PCoA plots showing beta diversity of samples collected fromM. fuscataswabs of the intestinal (blue), vaginal (red) or oral cavity (orange). The number of animals (n) used for each body site is indicated in parenthesis in the figure legend. (b) Phylum level abundance of bacteria isolated from the intestinal, vaginal or oral cavity ofM. fuscata(this work) orH. sapiens(leveraged from the HMP, available athttp://www.hmpdacc.org/). Each phylum is represented by a different colour in the phylogenetic tree. The total number of dams and juveniles from which microbiome characterization was derived were 50, with specimens from multiple body sites. Figure 1: Characterization of the Macaca fuscata microbiome. DNA was isolated from M. fuscata or H. sapiens swabs collected from the intestinal (anus, colorectal, and stool), vaginal or oral cavity. 16S rDNA sequencing was performed via the 454 FLXtitanium system and sequences were analysed using QIIME software. ( a ) PCoA plots showing beta diversity of samples collected from M. fuscata swabs of the intestinal (blue), vaginal (red) or oral cavity (orange). The number of animals ( n ) used for each body site is indicated in parenthesis in the figure legend. ( b ) Phylum level abundance of bacteria isolated from the intestinal, vaginal or oral cavity of M. fuscata (this work) or H. sapiens (leveraged from the HMP, available at http://www.hmpdacc.org/ ). Each phylum is represented by a different colour in the phylogenetic tree. The total number of dams and juveniles from which microbiome characterization was derived were 50, with specimens from multiple body sites. Full size image Next, we compared taxa at each body site with publicly available data from the Human Microbiome Project (HMP; hmpdacc.org). At the phylum level, intestinal taxa were similar and dominated by Bacteroidetes and Firmicutes ( Fig. 1b ). However, at the genus level, differences in Bacteroidetes were apparent. Specifically, the preponderance of Bacteroides in human and Prevotella in macaque is most likely a reflection of dietary differences. Bacteroides encodes enzymes for the digestion of saturated fats and animal-derived proteins more common in the Western diet [5] , while metabolic reconstructions in Prevotella are dominated by pathways for digestion of plant xylan and cellulose, which are more prevalent in the omnivorous diet of M. fuscata and of agrarian human populations, such as those in Burkina Faso [5] . Oral microbiota were similarly broadly akin at the phylum level, with the exception for a greater relative abundance of Fusobacteria in humans ( Fig. 1b ). Overall, the intestinal and oral microbial communities of M fuscata are similar to those of humans. The vaginal microbiome of M. fuscata contained less Lactobacillus than that of the human, was strikingly more diverse than humans and harboured taxa most often associated with the intestinal microbiome. While increased bacterial diversity in the human vaginal microbiome is associated with bacterial vaginosis [34] , [35] , other non-human primates (for example, baboons) harbour vaginal microbial diversity similar to what we observed in the healthy, non-gravid macaque [36] . Co-clustering of some vaginal and intestinal samples ( Fig. 1a ) suggests that these taxonomic abundance profiles in the macaque are most likely due to anatomic and differences in hygiene that result in faecal contamination. Diet primarily structures the intestinal microbiome ‘Obese’ microbiota have previously been implicated in the intestinal metabolic dysbiosis believed to promote host adiposity [1] , [15] , [21] , [22] , [23] . To assess the role of diet versus habitus in structuring the maternal gut microbiome, we maintained dams on a relative isocaloric diet consisting of high fat (36% fat from animal fat, fish oil and corn oil) or control chow (13% fat from soy bean oil) as previously reported [26] , [27] , [28] , [29] , [30] , [31] , [32] , [37] . In general, animals fed a control diet (CTD) remained lean while dams fed a high-fat diet (HFD) over at least 3 years either progressed to obesity (roughly two-thirds of our cohort; high-fat diet sensitive, HFDS) or remained lean (high-fat diet resistant, HFDR) [25] , [26] , [38] ( Supplementary Fig. 1a ). In addition to differences in weight gain, HFDS dams become insulin resistant while HFDR dams do not [25] . Despite this loss of sensitivity to insulin, we have not previously detected an increase in blood glucose levels as insulin resistance progresses [25] . Further metabolite analysis between HFDS and HFDR dams revealed differences between these two cohorts, including statistically significant increases in α-tocopherol, γ-tocopherol, glycine, aminomalonic acid and citric acid in HFDS dams when compared with HFDR and control cohorts; however, cholesterol is significantly increased in both HFDS and HFDR cohorts when compared with the control cohort [26] . Regardless of obesity and insulin resistance, HFDS (obese, insulin resistant) and HFDR (lean, insulin sensitive) dams clustered together and were distinct from CTD dams by PCoA ( P =0.001 by Permutational multivariate analysis of variance (PERMANOVA), Fig. 2a ). This finding was corroborated by measures of alpha diversity and species richness, which failed to detect a significant difference between HFDS and HFDR dams ( Supplementary Fig. 1b,c ). Interestingly, there are no apparent differences in the levels of inflammatory cytokines in the circulating plasma [37] that would explain differential clustering by virtue of diet. However, increases in total fatty acids (saturated, monosaturated, polyunsaturated and essential) and n-6 fatty acids have been reported for dams consuming a HFD [38] , which is a plausible explanation for why no differences are seen in the intestinal microbiome by habitus and insulin resistance. 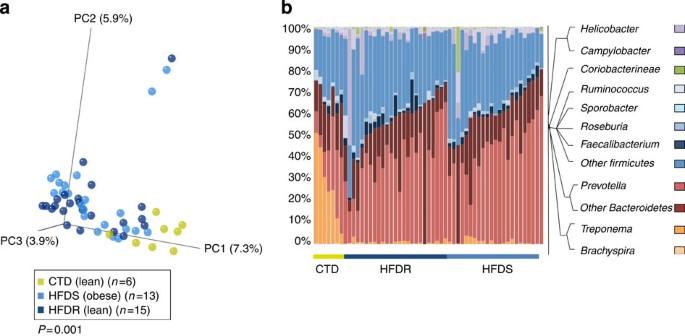Figure 2: Diet structures the intestinal microbiome ofMacaca fuscata. Intestinal samples were collected fromM. fuscatamaintained on an isocaloric diet consisting of either 13% fat (control diet) or 36% fat (high fat diet). DNA was isolated from intestinal contents and 16S rDNA pyrosequencing (454 FLXtitanium) was performed. Sequences were analysed using QIIME software. (a) PCoA plot demonstrating differential clustering of control diet (CTD, green), high-fat diet lean (HFDR, dark blue) or high-fat diet obese (HFDS, light blue) individuals. Individuals cluster significantly based on diet (P=0.001 by PERMANOVA). The number of animals in each category (n) is indicated in the parenthesis on the legend. (b) Graph demonstrating phylum abundance differences between control diet (CTD), high-fat diet lean (HFDR) and high-fat diet obese (HFDS) individuals. Legend to the right of the graph indicates the colour for each phyla of bacterium represented. Figure 2: Diet structures the intestinal microbiome of Macaca fuscata . Intestinal samples were collected from M. fuscata maintained on an isocaloric diet consisting of either 13% fat (control diet) or 36% fat (high fat diet). DNA was isolated from intestinal contents and 16S rDNA pyrosequencing (454 FLXtitanium) was performed. Sequences were analysed using QIIME software. ( a ) PCoA plot demonstrating differential clustering of control diet (CTD, green), high-fat diet lean (HFDR, dark blue) or high-fat diet obese (HFDS, light blue) individuals. Individuals cluster significantly based on diet ( P =0.001 by PERMANOVA). The number of animals in each category ( n ) is indicated in the parenthesis on the legend. ( b ) Graph demonstrating phylum abundance differences between control diet (CTD), high-fat diet lean (HFDR) and high-fat diet obese (HFDS) individuals. Legend to the right of the graph indicates the colour for each phyla of bacterium represented. Full size image Maintenance on the HFD through multiple pregnancies resulted in significant variation of intestinal taxa among dams with likely metabolic significance. While there were no significant variations in Firmicutes by virtue of neither maternal diet nor habitus (lean nor obese), dominance of Bacteroidetes and greatly decreased abundance of Spirochetes characterized the intestinal profile of the HFD-fed dams ( Figs 2b and 3b ). When we applied linear discriminate analysis to estimate effect size (LEfSe), providing a global view of the microbial shifts in association with dietary manipulation or maternal habitus ( Fig. 3a ), we found niche membership was structured by diet and occurred independently of sensitivity to the HFD (for example, independent of lean versus obese maternal phenotype). These shifts were primarily due to a great decrease of Treponema with corresponding increased relative abundance of Prevotella as revealed by Boruta feature selection ( Fig. 3b ). Treponema reads mapped primarily to T. berlinense , T. porcinum and T. parvum , none of which are known to be pathogenic in the intestinal environment [39] , [40] . Rather, it is of particular interest that the growth of these Treponema spp. is enhanced by carbohydrates, including galacturonic acid from plant pectin and other complex carbohydrates commonly found in corn and soy beans [39] , [40] . It is thus most plausible that diet components themselves conferred a growth advantage to Treponema spp. over Prevotella spp. in dams fed a control 13% fat diet. The intestinal microbiome from dams maintained on a CTD was similarly enriched for Sporobacter termitidis , a Firmicute first isolated from termites but also present in human intestinal microbiota, which synthesizes fatty acids from plant lignocellulose [41] , [42] . Lastly, Succinivibrio , a starch and cellulose fermenting genus of Gammaproteobacteria found in ruminants and rural African humans [43] , was paradoxically enriched in several dams in the HFD cohort. In these animals, Succinivibrio may have secured a niche by facilitating the establishment of a commensal or beneficial fermentation balance using intermediary metabolites from other microbes rather than dietary metabolites to grow [44] . 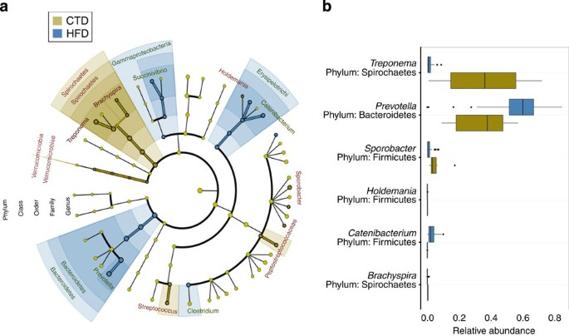Figure 3: Diet structures the intestinal microbiome ofMacaca fuscataat the genus level. Intestinal samples were collected fromM. fuscatamaintained on an isocaloric diet consisting of either 13% fat (control diet) or 36% fat (high fat diet). DNA was isolated from intestinal contents, and 16S rDNA pyrosequencing (454 FLXtitanium) was performed. Sequences were analysed using QIIME software. (a) Cladogram obtained from LEfSe analysis of 16S sequences. Green shaded areas indicate bacteria with a higher abundance in control diet fed animals (CTD), while blue shaded areas indicate bacteria with a higher abundance in animals fed a high-fat diet (HFD). (b) Relative abundance of bacterial genera between animals fed a control diet (CTD, green bars) or a high-fat diet (HFD, blue bars). Box plots demonstrate the distribution of data with the line in the middle of the box representing the median. The left of the median is indicative of the third quartile and the right is indicative of the first quartile. Lines to the right of the box are indicative of the 1.5 interquartile range of the lower quartile and lines to the left are indicative of the 1.5 interquartile range of the upper quartile. Dots represent outliers. Figure 3: Diet structures the intestinal microbiome of Macaca fuscata at the genus level. Intestinal samples were collected from M. fuscata maintained on an isocaloric diet consisting of either 13% fat (control diet) or 36% fat (high fat diet). DNA was isolated from intestinal contents, and 16S rDNA pyrosequencing (454 FLXtitanium) was performed. Sequences were analysed using QIIME software. ( a ) Cladogram obtained from LEfSe analysis of 16S sequences. Green shaded areas indicate bacteria with a higher abundance in control diet fed animals (CTD), while blue shaded areas indicate bacteria with a higher abundance in animals fed a high-fat diet (HFD). ( b ) Relative abundance of bacterial genera between animals fed a control diet (CTD, green bars) or a high-fat diet (HFD, blue bars). Box plots demonstrate the distribution of data with the line in the middle of the box representing the median. The left of the median is indicative of the third quartile and the right is indicative of the first quartile. Lines to the right of the box are indicative of the 1.5 interquartile range of the lower quartile and lines to the left are indicative of the 1.5 interquartile range of the upper quartile. Dots represent outliers. Full size image Maternal diet structures the offspring microbiome Given the high heritability, lack of readily identifiable genetic contributions, and uncertain origins of microbial dysbioses associated with diseases such as type 2 diabetes mellitus and inflammatory bowel disease [10] , [11] , [12] , we sought to determine whether changes in maternal microbiota associated with a HFD could be detected in the post-weaning microbiome profile of their offspring. To test the hypothesis that the maternal diet structures a dysbiotic intestinal microbiome later in life, M. fuscata dams were maintained on their designated diet (CTD versus HFD) over the course of gestation and through lactation. Offspring were delivered vaginally and breastfed exclusively until weaning (6–7 months), when they were either maintained or switched to the other diet formulation. This enabled comparison of the resultant offspring’s microbiome based on the combination of maternal gestation/lactation diet (CTD or HFD) with the juvenile post-weaning diet (CTD or HFD). Offspring were not cross-fostered since these types of studies are prone to failure [45] , which results in the continual exposure of offspring to n-3 fatty acids via breast milk [38] . However, this design provides a translational approach for comparison with human microbiome development. Our study design resulted in cohorts of animals with a gestation/lactation control diet/post-weaning control diet (CTD/CTD), a gestation/lactation high-fat diet/post-weaning high-fat diet (HFD/HFD), a gestation/lactation high-fat diet/post-weaning control diet (HFD/CTD) or a gestation/lactation control diet/post-weaning high-fat diet (CTD/HFD). While the average weight at the time of measure was similar among the four juvenile cohorts over the first year of life, we did see that weight gain between the groups was significantly different ( Supplementary Fig. 2a ). Juveniles were maintained on the post-weaning diet for ~6 months, or until 1 year of age, which is the approximate developmental equivalent in humans for the emergence of adult microbiota [3] , [46] . To confirm that juveniles harboured non-gravid, healthy, adult-like intestinal microbiota and to examine the ability of the post-weaning CTD to correct maternally inherited dysbioses, we performed PCoA of maternal and juvenile microbiome samples ( Fig. 4a ). Significant co-clustering of samples by maternal or post-weaning diet, rather than age, indicates that, by the end of the first year, the intestinal M. fuscata microbiome has reached relative stability ( P =0.001 by PERMANOVA, based on the post-weaning diet). Next, we investigated the impact of gestation/lactation and/or post-weaning HFD exposure diet on the trajectory of the offspring microbiome by examining eight maternal-fetal pairs (connected by solid lines in Fig. 4a ). We found that the post-weaning diet, rather than maternal diet, was largely predictive of clustering ( Fig. 4a ). In agreement, CTD/HFD juveniles clustered with HFD adults and HFD/CTD juveniles clustered with CTD adults ( Fig. 4a ). However, the tightest and most significant dysbiosis was observed among offspring who experienced a HFD during gestation/lactation followed by a HFD post-weaning ( P =0.001 by PERMANOVA, Fig. 4b ). Similarly, weaning onto a CTD after intrauterine exposure to a HFD failed to entirely correct the resultant intestinal dysbiosis ( P =0.016 by PERMANOVA, Fig. 4c ). This failure to correct the dysbiosis may not only be due to gestational HFD exposure but also be due the short exposure of the CTD post-weaning. However, studies examining the stabilization of the infant microbiome have found that this stabilization is achieved by 3 years of age [3] , [46] , which should be the developmental equivalent in our model system. Further, it was recently shown by David et al. [24] that the intestinal microbiome can be altered drastically in a remarkably short period of time. Another possibility is the stress of a new environment may prevent complete correction of dysbiosis caused by the maternal diet. However, we feel that this is an unlikely possibility since juveniles should be well adjusted to their new environment at the time of analysis. Therefore, based on these previous studies, our data suggest that exposure to a HFD during gestation is the most likely culprit for persistent alterations in the microbiome described here. Altogether, these findings indicate that, while the post-weaning diet is capable of partially correcting maternal diet-driven dysbioses, persistent differences in the offspring intestinal microbiome community observed are most likely due to dietary exposure during gestation and breastfeeding. This is both consistent with and greatly expands on our work and those of others [24] , [25] , [26] , [27] , [28] , [29] , [30] , [31] , [32] , [33] , [34] on the developmental origins of disease, which collectively suggest a period of unique susceptibility to metabolic programming during in utero and early postnatal environment. 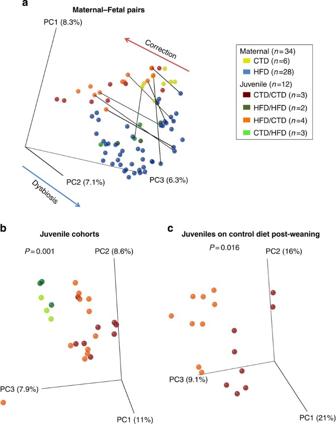Figure 4: Maternal and juvenile dietary manipulations synergistically alter the offspring microbiome. M. fuscataoffspring were vaginally delivered to mothers consuming a control (CTD) or high-fat diet (HFD). Infants consumed the maternal diet until weaning when they were either maintained on the maternal diet (control cohort) or switched to the opposing diet (crossover cohort). At 1 year of age, juveniles were killed and DNA was isolated from intestinal samples. DNA was subjected to 16S rDNA pyrosequencing, and sequences were analysed using QIIME. Mothers consuming a high-fat diet are indicated by dark blue (HFD), and control diet mothers are indicated by yellow (CTD). Juveniles are designated based on the maternal/post-wean diets; that is, CTD/HFD indicates a juvenile that was born to a dam consuming a control diet and switched to a high-fat diet post-weaning. Red represents juveniles on a control diet/control diet (CTD/CTD), dark green indicates juveniles on a high-fat diet/high fat diet (HFD/HFD), orange indicates juveniles on a high-fat diet/control diet (HFD/CTD) and light green indicates juveniles on a control diet/high-fat diet (CTD/HFD). Lines connect maternal-fetal pairs. The number of dams or juveniles in each cohort (n) is indicated in the parenthesis on the legend. (a) PCoA of intestinal samples from maternal-fetal pairs. (b) PCoA of intestinal samples from all juvenile cohorts. Juveniles exposed to a high-fat diet post-weaning significantly clustered (P=0.001 by PERMANOVA) when compared with juveniles exposed to a control diet post-weaning. (c) PCoA of intestinal samples from juveniles maintained on a control diet post-weaning. Juveniles exposed to a high-fat diet pre-weaning significantly clustered (P=0.016 by PERMANOVA) when compared with juveniles exposed to a control diet post-weaning. Figure 4: Maternal and juvenile dietary manipulations synergistically alter the offspring microbiome. M. fuscata offspring were vaginally delivered to mothers consuming a control (CTD) or high-fat diet (HFD). Infants consumed the maternal diet until weaning when they were either maintained on the maternal diet (control cohort) or switched to the opposing diet (crossover cohort). At 1 year of age, juveniles were killed and DNA was isolated from intestinal samples. DNA was subjected to 16S rDNA pyrosequencing, and sequences were analysed using QIIME. Mothers consuming a high-fat diet are indicated by dark blue (HFD), and control diet mothers are indicated by yellow (CTD). Juveniles are designated based on the maternal/post-wean diets; that is, CTD/HFD indicates a juvenile that was born to a dam consuming a control diet and switched to a high-fat diet post-weaning. Red represents juveniles on a control diet/control diet (CTD/CTD), dark green indicates juveniles on a high-fat diet/high fat diet (HFD/HFD), orange indicates juveniles on a high-fat diet/control diet (HFD/CTD) and light green indicates juveniles on a control diet/high-fat diet (CTD/HFD). Lines connect maternal-fetal pairs. The number of dams or juveniles in each cohort ( n ) is indicated in the parenthesis on the legend. ( a ) PCoA of intestinal samples from maternal-fetal pairs. ( b ) PCoA of intestinal samples from all juvenile cohorts. Juveniles exposed to a high-fat diet post-weaning significantly clustered ( P =0.001 by PERMANOVA) when compared with juveniles exposed to a control diet post-weaning. ( c ) PCoA of intestinal samples from juveniles maintained on a control diet post-weaning. Juveniles exposed to a high-fat diet pre-weaning significantly clustered ( P =0.016 by PERMANOVA) when compared with juveniles exposed to a control diet post-weaning. Full size image Given the persistence of the effect of maternal HFD exposure on the resultant offspring intestinal taxa, we sought to determine which genus members and taxonomic metabolic pathways or carriage patterns were driving these findings. Boruta feature selection of 16S-derived metagenomic data revealed maternal HFD-driven depletion of Proteobacteria, specifically the Epsilonproteobacteria Campylobacter spp. and Helicobacter spp, alongside the enrichment of the Firmicutes Ruminococcus and Dialister ( Fig. 5a ). When we further interrogated the 16S-derived metagenomic data at the genus level, we found that Campylobacter spp were decreased in offspring following any exposure to a HFD either during gestation/lactation or post-weaning ( Figs 5b and 6 ). As in our maternal CTD cohort ( Figs 2b and 3b ), juveniles maintained on a CTD post-weaning likewise carried increased Treponema ( Figs 5 and 6 ). As gross measures of community diversity, analysis of the offspring intestinal taxa demonstrated decreased measures of species richness ( Supplementary Fig. 2b ) and diversity ( Supplementary Fig. 2c ) with any measure of high-fat dietary exposure; this observation was confirmed by LEfSe ( Supplementary Fig. 2d ). 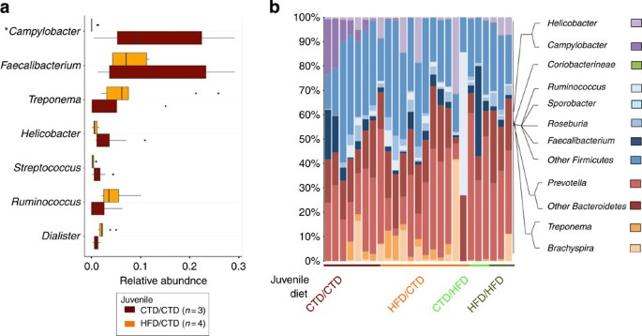Figure 5: Exposure to a maternal high-fat diet persistently alters the offsprings intestinal microbiome with significant depletion of Proteobacteria, including Campylobacter spp. M. fuscataoffspring were vaginally delivered to mothers consuming a control (CTD) or high-fat diet (HFD). Infants consumed the maternal diet until weaning when they were either maintained on the maternal diet (control cohort) or switched to the opposing diet (crossover cohort). At 1 year of age, juveniles were killed and DNA was isolated from intestinal samples. DNA was subjected to 16S rDNA pyrosequencing, and sequences were analysed using QIIME. Juveniles are designated based on the maternal/post-wean diets; that is, CTD/HFD indicates a juvenile that was born to a dam consuming a control diet and switched to a high fat diet post-weaning. Red colour represents juveniles on a control diet/control diet (CTD/CTD), dark green indicates juveniles on a high-fat diet/high fat diet (HFD/HFD), orange indicates juveniles on a high-fat diet/control diet (HFD/CTD) and light green indicates juveniles on a control diet/high-fat diet (CTD/HFD). (a) Relative abundance of bacterial genera in intestinal samples of juveniles maintained on a control diet post-weaning. Juveniles are designated based on the maternal/post-wean diet. Box plots show the distribution of data, with the line in the middle of the box representing the median. The left of the median is indicative of the third quartile and the right is indicative of the first quartile. Lines to the right of the box are indicative of the 1.5 interquartile range of the lower quartile and lines to the left are indicative of the 1.5 interquartile range of the upper quartile. Dots represent outliers. The asterisk byCampylobacterindicates a statistically significant difference (P<0.05 byt-test) between CTD/CTD and HFD/CTD juveniles. (b) Graph representing the most abundant bacterial genera present in intestinal samples of differential juvenile cohorts. Juveniles are grouped based on maternal/post-wean diet as indicated by the line below the chart. Phylogenetic tree designates the genus represented by each colour. Figure 5: Exposure to a maternal high-fat diet persistently alters the offsprings intestinal microbiome with significant depletion of Proteobacteria, including Campylobacter spp. M. fuscata offspring were vaginally delivered to mothers consuming a control (CTD) or high-fat diet (HFD). Infants consumed the maternal diet until weaning when they were either maintained on the maternal diet (control cohort) or switched to the opposing diet (crossover cohort). At 1 year of age, juveniles were killed and DNA was isolated from intestinal samples. DNA was subjected to 16S rDNA pyrosequencing, and sequences were analysed using QIIME. Juveniles are designated based on the maternal/post-wean diets; that is, CTD/HFD indicates a juvenile that was born to a dam consuming a control diet and switched to a high fat diet post-weaning. Red colour represents juveniles on a control diet/control diet (CTD/CTD), dark green indicates juveniles on a high-fat diet/high fat diet (HFD/HFD), orange indicates juveniles on a high-fat diet/control diet (HFD/CTD) and light green indicates juveniles on a control diet/high-fat diet (CTD/HFD). ( a ) Relative abundance of bacterial genera in intestinal samples of juveniles maintained on a control diet post-weaning. Juveniles are designated based on the maternal/post-wean diet. Box plots show the distribution of data, with the line in the middle of the box representing the median. The left of the median is indicative of the third quartile and the right is indicative of the first quartile. Lines to the right of the box are indicative of the 1.5 interquartile range of the lower quartile and lines to the left are indicative of the 1.5 interquartile range of the upper quartile. Dots represent outliers. The asterisk by Campylobacter indicates a statistically significant difference ( P <0.05 by t -test) between CTD/CTD and HFD/CTD juveniles. ( b ) Graph representing the most abundant bacterial genera present in intestinal samples of differential juvenile cohorts. Juveniles are grouped based on maternal/post-wean diet as indicated by the line below the chart. Phylogenetic tree designates the genus represented by each colour. 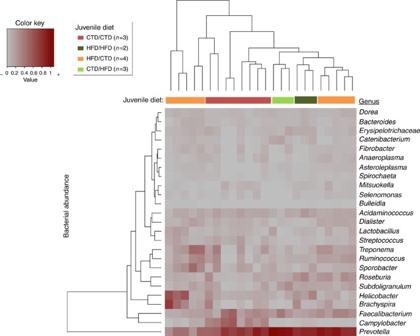Figure 6: Genus level projections of bacterial abundance in juvenile offspring demonstrating persistent impact of a maternal high fat diet. Heat map indicating genus-level changes betweenM. fuscataconsuming either a control or high-fat diet during gestation/lactation and/or post-weaning. Relative abundance of each genus is indicated by a gradient of colour from grey (low abundance) to red (high abundance). Heat map generated using Manhattan distance and hierarchical clustering is based on average linkage. Legend above heat map indicates the maternal and post-wean diet of each juvenile represented. On the basis of the dendrogram, a cluster of samples from juveniles consuming a control/control diet is observed due to higherCampylobacterabundance. The number of juveniles (n) in each cohort is indicated in parenthesis in the figure legend. Full size image Figure 6: Genus level projections of bacterial abundance in juvenile offspring demonstrating persistent impact of a maternal high fat diet. Heat map indicating genus-level changes between M. fuscata consuming either a control or high-fat diet during gestation/lactation and/or post-weaning. Relative abundance of each genus is indicated by a gradient of colour from grey (low abundance) to red (high abundance). Heat map generated using Manhattan distance and hierarchical clustering is based on average linkage. Legend above heat map indicates the maternal and post-wean diet of each juvenile represented. On the basis of the dendrogram, a cluster of samples from juveniles consuming a control/control diet is observed due to higher Campylobacter abundance. The number of juveniles ( n ) in each cohort is indicated in parenthesis in the figure legend. Full size image Obese microbiota may confer increased dietary energy-harvesting capacity in hosts consuming a HFDthrough global alterations in the enzymatic capacity of the microbiome. To test this hypothesis, we performed phylogenetic investigation of communities by reconstruction of unobserved states (PICRUSt) of microbiota sequences obtained from 16S pyrosequencing of juvenile cohorts maintained on a CTD post-weaning. This analysis allowed us to determine whether diet altered the metabolic capacity and overarching gene carriage patterns in offspring. Functional composition profiles based on the Kyoto encyclopedia of genes and genomes (KEGG, http://www.ncbi.nlm.nih.gov/pubmed/22080510 ) were generated by PICRUSt, and these functional profiles were then correlated to the genus level relative abundance of selected bacterium that were identified through Boruta feature selection and LEfSe ( Fig. 7 ). In addition to changes in the abundance of Campylobacter depending on the gestation/lactation diet, we observed that any residual Campylobacter in HFD/CTD juveniles correlate positively with pathways involved in amino-acid metabolism, carbohydrate metabolism and lipid metabolism. These results are similar to those seen in mice that are either genetically altered to induce obesity or are transplanted with ‘obese’ mirobiota [1] , [9] . In agreement, the presence of Campylobacter spp in CTD/CTD juveniles negatively correlates with some of the same metabolic pathways including those involved in lipid metabolism. In particular, we found that arachidonic-acid metabolism negatively correlated with the presence of Campylobacter in CTD/CTD juveniles. In contrast to changes in metabolic pathways associated with Campylobacter carriage, the genus Ruminococcus displayed a positive correlation with these pathways regardless of diet ( Fig. 7 ). Thus, these correlations may aid in the identification of bacteria involved in metabolic pathways that promote or suppress the development of adipose tissue. Taken together, these data further demonstrate the longitudinal impact of the gestation/lactation diet on juveniles. Consequently, microbial shifts resulting from maternal dietary habits during gestation likely influence the metabolic processes of offspring. 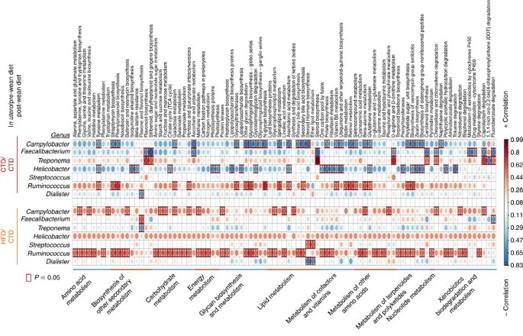Figure 7: A maternal high fat diet persistently and significantly alters functional microbial metabolic pathways among juvenile offspring. Bacterial metabolic pathways of juveniles differ based on maternal gestational diet. Correlations between a PICRUSt-generated functional profile and a QIIME-generated genus level bacterial abundance were calculated and plotted subject to the gestation/lactation diet between juveniles exposed to a maternal control or high-fat diet. Only genera identified by Boruta feature selection and LEfSe as significantly different between juveniles exposed to a control versus high-fat gestational/lactational diet are shown in the figure. Metabolic pathway designations are indicated at the bottom of the graph. The upper part of the graph represents juveniles exposed to a control diet gestation/lactation (CTD/CTD, red bar) while the lower part represents juveniles exposed to a high-fat diet during gestation/lactation (HFD/CTD, orange bar). The shading intensity of the bubble, along with size, is indicative of the Kendall rank correlation coefficient between matrices. Blue designates a positive correlation while orange/red designates a negative correlation. Red squares surrounding a bubble are indicative of a significantP-value≤0.05 by Kendall’s test;n=3 juveniles exposed to control/control diet, andn=4 for juveniles exposed to high-fat diet/control diet. Figure 7: A maternal high fat diet persistently and significantly alters functional microbial metabolic pathways among juvenile offspring. Bacterial metabolic pathways of juveniles differ based on maternal gestational diet. Correlations between a PICRUSt-generated functional profile and a QIIME-generated genus level bacterial abundance were calculated and plotted subject to the gestation/lactation diet between juveniles exposed to a maternal control or high-fat diet. Only genera identified by Boruta feature selection and LEfSe as significantly different between juveniles exposed to a control versus high-fat gestational/lactational diet are shown in the figure. Metabolic pathway designations are indicated at the bottom of the graph. The upper part of the graph represents juveniles exposed to a control diet gestation/lactation (CTD/CTD, red bar) while the lower part represents juveniles exposed to a high-fat diet during gestation/lactation (HFD/CTD, orange bar). The shading intensity of the bubble, along with size, is indicative of the Kendall rank correlation coefficient between matrices. Blue designates a positive correlation while orange/red designates a negative correlation. Red squares surrounding a bubble are indicative of a significant P -value≤0.05 by Kendall’s test; n =3 juveniles exposed to control/control diet, and n =4 for juveniles exposed to high-fat diet/control diet. Full size image HFD diminishes Campylobacter in offspring 16S rRNA sequencing indicated juveniles exposed to a gestation/lactation or post-weaning HFD demonstrated markedly decreased carriage of the Epsilonproteobacteria genus Campylobacter when compared with the juvenile cohort exposed to CTD both during gestation/lactation and post weaning (CTD/CTD). To validate this observation, we confirmed the carriage of Campylobacter at the genus level in the stool of the CTD/CTD cohort and the reduction of Campylobacter in the stool of juvenile cohorts exposed to the HFD, either during gestation/lactation or post-weaning ( Fig. 8 ). As none of our juvenile cohorts displayed signs or symptoms of Campylobacteriosis, we conclude the Campylobacter spp. present in the CTD/CTD cohort was commensal in nature, as previously shown [47] , [48] . These data confirm through culture-independent methods that the maternal dietary habits during gestation are able to persistently alter the offspring microbiota. 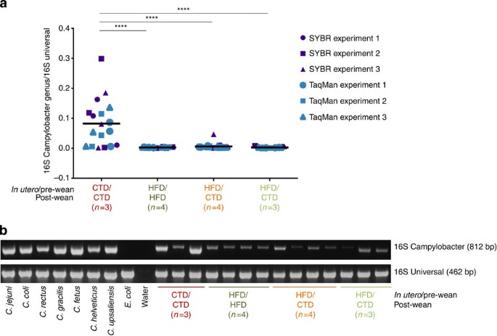Figure 8: Exposure to a high-fat diet diminishes the presence ofCampylobacter. M. fuscatawas vaginally birthed to mothers consuming a control or high-fat diet. Infants consumed the maternal diet until weaning when they were either maintained on the maternal diet (control cohort) or switched to the opposing diet (crossover cohort). At 1 year of age, animals were killed and DNA was isolated from the stool. DNA was subjected to PCR amplification for both universal 16S rRNA and forCampylobacter16S rRNA genes. The number of juveniles (n) in each cohort is indicated in parenthesis in the figure legend. (a) Quantitative real-time PCR (qPCR) analysis of stool isolated from juvenile cohorts designated by maternal/post-wean diet. DNA was amplified for universal andCampylobacter16S rRNA genes using both TaqMan and SYBR qPCR assays. The presence ofCampylobacter16S rRNA was normalized to total universal 16S rRNA presence to provide relative abundance. Each qPCR assay (TaqMan or SYBR) was repeated in three individual assays. Results were pooled and statistical analysis was performed using a one-way ANOVA (**P<0.05). Line represents the mean. (b) PCR amplification ofCampylobacter16S rDNA (top, 812 bp) or universal 16S rDNA (bottom, 462 bp). PCR products were run on a 3% agarose gel containing ethidium bromide. Full gel can be seen inSupplementary Fig. 3. Figure 8: Exposure to a high-fat diet diminishes the presence of Campylobacter . M. fuscata was vaginally birthed to mothers consuming a control or high-fat diet. Infants consumed the maternal diet until weaning when they were either maintained on the maternal diet (control cohort) or switched to the opposing diet (crossover cohort). At 1 year of age, animals were killed and DNA was isolated from the stool. DNA was subjected to PCR amplification for both universal 16S rRNA and for Campylobacter 16S rRNA genes. The number of juveniles ( n ) in each cohort is indicated in parenthesis in the figure legend. ( a ) Quantitative real-time PCR (qPCR) analysis of stool isolated from juvenile cohorts designated by maternal/post-wean diet. DNA was amplified for universal and Campylobacter 16S rRNA genes using both TaqMan and SYBR qPCR assays. The presence of Campylobacter 16S rRNA was normalized to total universal 16S rRNA presence to provide relative abundance. Each qPCR assay (TaqMan or SYBR) was repeated in three individual assays. Results were pooled and statistical analysis was performed using a one-way ANOVA (** P <0.05). Line represents the mean. ( b ) PCR amplification of Campylobacter 16S rDNA (top, 812 bp) or universal 16S rDNA (bottom, 462 bp). PCR products were run on a 3% agarose gel containing ethidium bromide. Full gel can be seen in Supplementary Fig. 3 . Full size image In the present study, diet markedly altered the intestinal microbiome of mothers and their offspring at 1 year of age. Maintenance on the HFD through multiple pregnancies resulted in significant variation in intestinal taxa among dams with likely metabolic significance. While there were no significant variations in Firmicutes by virtue of either maternal diet or habitus (lean nor obese), the dominance of Bacteroidetes and the absence of Spirochetes dominated the intestinal profile of the HFD-fed dams. These shifts were primarily due to a great decrease of Treponema and increased relative abundance of Prevotella . In our primate model of maternal obesity, the diets are relatively isocaloric but the fat content varies from 13 to 36% by virtue of the fat constituents (13% control chow derived from soy bean oil versus 36% fat from animal fat, fish oil and corn oil) [27] , [28] , [30] . It is therefore of interest that microbes dependent on carbohydrates ( Treponema spp) are able to synthesize fatty acids from plant cellulose ( Sporobacter termitidis ), or starch and cellulose-fermenting bacteria (Gammaproteobacter Succinivibrio ) are paradoxically enriched not by habitus but rather by maternal diet [39] , [40] , [41] , [44] . Moreover, the relative abundance of these bacterial species does not significantly vary in either lean or obese dams when fed a HFD. Our observations collectively challenge the notion that there is an inherently ‘obesogenic’ microbiome and rather support emerging data from mice and humans suggesting a transmissible and modifiable interaction between diet and microbial community that influence host biology (adiposity) [9] , [24] . Our data demonstrating a role for the maternal diet, rather than maternal obesity per se , in shaping the offspring gut microbiome at 1 year of age is consistent with our prior findings on its impact on the fetal epigenome [27] , [28] , [30] . Although we have previously seen that diet reversal post-weaning can rescue the expression of genes involved in the circadian pathway [27] , [28] , diet reversal post-weaning does not correct for all in utero changes to the fetal epigenome [30] . Here, we describe another persistent change in offspring due to maternal diet with the genus Campylobacter being diminished based on the maternal diet. In addition to the implications for the role of the microbiota in changing epigenetics, or vice versa, these persistent alterations in the microbiome may promote the behavioural changes in anxiety that have previously been described [32] . Altogether, these data reveal potential pathways involved in the crosstalk between biological systems. Our findings presented in Figs 4 and 5 , and Supplementary Fig. 2 significantly extend the observations of Le Chatelier et al. [8] and Cotillard et al. [49] In their human population-based metagenomic studies, they demonstrate that low and high gene count tracks with bacterial richness, which is in turn associated with the upper quartile of their study population characterized by increased adiposity, insulin resistance, dyslipidemia and markers of inflammation [8] , [49] . In addition, dietary intervention restored species richness in low gene count individuals [49] . In our primate study, we are able to leverage nearly a decade of experience delineating the disparate resultant phenotype, which identified our HFDR (lean) and HFDS (obese) dams, to describe the attributable weighted impact of a caloric dense diet. When we delved deeper and correlated bacterium with KEGG metabolic pathways, we found trends in our juveniles exposed to a HFD during gestation/lactation that were similar to previous studies demonstrating that amino-acid metabolism, carbohydrate metabolism and lipid metabolism were upregulated in obese mice [1] , [9] . Despite the persistent changes we detected in juveniles exposed to HFD, collectively our findings, and those of others, [8] , [9] , [24] , [49] should provide a note of optimism as it appears that diet, rather than obesity per se , is the greater arbiter of the intestinal microbiome. This notion is consistent with multiple studies demonstrating resultant shifts in the intestinal microbiome following dietary modification [1] , [22] , [23] . The loss of a presumptive commensal genus [47] , [48] , Campylobacter , from the intestinal microbiome in offspring is particularly intriguing when considered from the perspective of a microbial evolutionary ecologist. Campylobacter spp., include several human pathogens, such as C. jejuni, which mediates gastroenteritis, is an antecedent to Guillain-Barre syndrome and has previously been associated with increased incidence of inflammatory bowel disease and the post-infective development of celiac disease [50] , [51] . We find it notable that among HFD naive offspring, it is an apparent commensal genus as none of our offspring manifest any symptoms of gastric illness. Of note, offspring utilized in this study were co-housed at some juncture to achieve a combinatorial set of post-weaning dietary exposures. Thus, at one interval or another, CTD/CTD juveniles were co-housed with HFD/CTD and/or CTD/HFD juveniles, which allowed for exposure of HFD/CTD and CTD/HFD juveniles to Campylobacter . Our findings suggest that the maternal diet has the capacity to persistently alter intestinal commensal taxa in the offspring, in this case Campylobacter spp. By extension, it is possible that reintroduction of a previously commensal bacterial species later in life may result in intestinal dysbiosis and subsequent host pathology. Intriguingly, the genus Helicobacter has been similarly described to be a previous commensal organism that now is pathogenic [52] . Both Campylobacter and Helicobacter are part of the Epsilonbacteria class of the phylum Proteobacteria. Recently, H. pylori has been correlated with a decreased incidence of asthma and allergy, and has been shown to improve glucose homeostasis in mice [53] , [54] , [55] . Thus, it seems plausible that commensal Epsilonproteobacteria may provide protection from obesity-associated metabolic disorders. In summary, our data continue to support the idea that diet, rather than habitus, most likely drives ‘dysbiosis’ in primates and suggests that gut ecology may be structured across generations by multiple modalities, including the maternal diet. Before the advent of farming and cultivation, Homo sapiens were a nomadic culture whose diet consisted primarily of vegetation and leaner meats rather than high-fat animal products. However, the advent of farming and animal husbandry resulted in significantly increased fat intake, which has remained a staple of the Western diet. Drastic changes are seen in the intestinal microbiome between individuals in developing versus developed countries [5] , [19] . These key changes in the diet of Homo sapiens , along with the data presented here, may help to explain the depletion of Camplyobacter from the human intestinal microbiome, and likewise suggest short-term dietary manipulations combined with traditional antibiotics may represent a novel approach to the treatment of acute gastroenteric disease mediated by Campylobacter [52] . Altogether, our data suggest that a relatively stable adult microbiome is born out of a labile infant microbiome, which in primates is structured by the maternal and post-weaning diet. These findings have likely implications not only for individual and population-based disease later in life but also potentially for the evolution of human microbial ecology. Experimental design The use of M. fusata by our consortium of investigators has been previously described [26] , [27] , [28] , [29] , [30] , [31] . In brief, animals were socially housed (4–9 females and 1–2 males per group) within indoor/outdoor enclosures at the Oregon National Primate Research Center (ONPRC) and in accordance with the institutional animal care and use committees (IACUC) at both Baylor College of Medicine and ONPRC. Animals were on an isocaloric diet and were either fed a CTD of standard chow (Monkey Diet no. 5000; Purina Mills Co., St Louis, MO) consisting of 13% fat from soya bean oil or HFD (TAD Primate Diet 5LOP, Test Diet, Richmond, IN) consisting of 36% fat from lard, butter, animal fat and safflower oil that is additionally supplemented with calorically dense treats (consisting of Glaxo powder/TAD pellets, peanut butter, honey, banana and cornstarch). Animals bred naturally, and offspring (both male and female) were maintained on a similar diet as their mothers until weaning (6–7 months) when the offspring either became part of the control cohort (maintaining the same diet as their mothers’) or the crossover cohort (switching the diet from their mothers’). CTD or HFD cohorts were designated randomly. Animals were housed socially and based on diet. More specifically, since juveniles exposed to CTD/CTD or HFD/HFD did not change diets, these animals maintained housing with others on the CTD or HFD, respectively; however, CTD/HFD and HFD/CTD juveniles switched housing on weaning to accommodate their crossover diet. This resulted in the exposure of all juvenile cohorts to the intestinal microbiome based on CTD or HFD. Specifically, for the CTD/HFD juvenile cohorts, these animals were housed with CTD animals until weaning, when they were then cohoused with HFD animals. Conversely, for HFD/CTD juvenile cohorts, these animals were housed with HFD animals until weaning when they were housed with CTD animals. In addition, animals utilized in this study were not treated with antibiotics and had no gross evidence of malabsoprtion or chronic diarrhea. Therefore, dysbiosis detected in the microbiome are solely due to differences in diet. At 1 year of age, juveniles were killed by anaesthetizing with sodium pentobarbital before exsanguination. Sequencing of the microbiome Samples from the gastrointestinal tract (stool, ascending colon, anus), vaginal or oral cavity were collected, and DNA was isolated via the Powersoil DNA Isolation Kit (Mo Bio Laboratories, Carlsbad, CA). Intestinal samples were collected from the last stool, contents of the luminal side of the ascending colon, and by inserting a cotton swab into anus after necropsy. Oral and vaginal samples were collected by swabbing the body site. After DNA extraction, 16S rDNA of bacteria was amplified and barcodes attached for sample identification using V3V5 primers before 454 sequencing; the resulting sequences were analysed using quantitative insights into microbial ecology (QIIME) software [56] . The V3V5 primer sequences, with barcodes in lower case letters, are as follows: 5′-cctatcccctgtgtgccttggcagtctcaGCCTACGGGAGGCAGCAG-3′ (forward B-354F primer) and 5′-ccatctcatccctgcgtgtctccgactcagNNNNNCCGTCAATTCMTTTRAGT-3′ (reverse A-926R primer). 16S data analysis Preprocessing involved removing reads lacking a barcode or primer sequencing, and then removing reads with length less than 200 nucleotides and reads with minimum average quality less than 20. AmpliconNoise [57] was used to correct for errors introduced in PCR and pyrosequencing, as well as removing chimeric sequences. The flowgram distance was calculated first and hierarchical clustered with complete linkage. Then expectation-maximization algorithm was used to remove pyrosequencing noise and reads were further truncated to 400 base pairs. PCR error was calculated between sequences and clustered to provide as input to SeqNoise. PCR errors were subsequently removed by SeqNoise step. Primers and barcodes were excised from de-noised sequences. Finally, de-noised sequences were further clustered by means of complete linkage clustering into operational taxonomic units (OTUs) at the 97% similarity level through AmpliconNoise. OTUs appeared in <5% of samples were removed from OTU table. Each sequence, as well as de-noised OTU, was classified down to genus level using RDP classifier v2.2 (re-trained using the release Feb 4, 2011 of the GreenGenes taxonomy) [58] . The taxonomic assignment of each sequence was truncated at the most specific taxonomic level with a confidence score of at least 85%. Microbial diversity was evaluated within samples (alpha diversity) or between samples (beta diversity) on the OTU table. Alpha diversity measurements were performed using R package BiodiversityR. Plots were generated and exported for species richness and Renyi’s diversity indices. Beta diversity was evaluated with both non-phylogenetic (Canberra) and phylogenetic (Unifrac) distance [59] . The distance matrices were then served as inputs for PCoA and significance tests. PCoA was used in exploration of potential factors that might explain the groupings of similar communities. Statistical significance of groupings among samples over distance matrices were tested with PERMANOVA through QIIME. The significant taxa with differentiating clusters were identified by Boruta feature selection through R package Boruta [60] . LEfSe was also used to detect significant features. LEfSe combines the statistical test (Kurskal–Wallis test, pairwise Wilcoxon test) with linear discriminate analysis for feature selection and ranks feature by effect size [61] . The alpha value employed for the factorial Kruskal–Wallies test is 0.05. The threshold employed on the logarithmic LDA score for discriminative feature is 2.0. For bacterial metabolic activity abundance, as defined by the Kyoto encyclopedia of genes and genomes (KEGG), these data were generated by PICRUSt (the phylogenetic investigation of communities by reconstruction of unobserved states) [62] using closed-reference OTUs picked by QIIME over the same set of sequences. The correlation matrix between functional profile and genus level abundance was calculated and plotted in R. Quantitative PCR DNA isolated from stool samples from M. fuscata was subjected to quantitative real-time PCR (qPCR) for universal 16S rRNA and campylobacter genus specific 16S rRNA using Taqman probes (Molecular Probes, Grand Island, NY). For the universal 16S rRNA qPCR, the primer and probe sequences were [63] , [64] : 5′-TCCTACGGGAGGCAGCAGT-3′ (forward primer 16SuniversalFor), 5′-GGACTACCAGGGTATCTAATCCTGTT-3′ (reverse primer 916SuniversalRev), and 6-carboxyfluorescein(FAM)-5′- CGTATTACCGCGGCTGCTGGCAC-3′-tetramethylrhodamine(TAMRA) (probe 16Suniversalprobe). For the Campylobacter genus specific 16S rRNA qPCR, the primer and probe sequences were [47] , [65] 5′-GAAGGTGTGGACGACGTCAA-3′ (forward primer 16Scampy_genusF2), 5′-ATATGCCATTGTAGCACGTGTGT-3′ (reverse primer 16Scampy_genusR3), and 5′-ATCATGGCCCTTATGC-3′ (16Scampy_genus_probe, minor groove binder MGB ). The annealing temperature for the qPCR was set at 60 °C and ran for 45 cycles. Data were analysed using StepOne software (Applied Biosystems, Life Technologies, Grand Island, NY). For SYBR green qPCR assays, 16SuniversalFor and 16SuniversalRev primers were used for detection of universal 16S rDNA. For Campylobacter genus, we used either the primer set 16Scampy_genusF2 and 16Scampy_genusR3 or the primer set 16Scampy_genusF1 (5′-CACGTGCTACAATGGCATAT-3′) and 16Scampy_genusR2 (5′-GGCTTCATGSWSTCGAGTT-3′). Both universal and Campylobacter 16S rDNAs were amplified with a 60 °C annealing temperature. The presence of Campylobacter 16S rDNA was normalized to universal 16S rDNA expression. Statistical analysis was performed using one-way ANOVA via GraphPad Prism software (La Jolla, CA). In addition, DNA isolated from M. fusata was also subjected to PCR amplification for the Campylobacter genus and the universal 16S rDNA as previously described [47] , [65] . The primers used for the Campylobacter genus-specific PCR were C412F 5′- GGATGACACTTTTCGGAGC -3′ and C1288R 5′- GGATGACACTTTTCGGAGC-3′. These primers generated an 812 bp product using 28 cycles of PCR amplification at 94 °C for 1 min, 55 °C for 1 min and 72 °C for 1 min. Universal 16S rDNA was amplified using the primers described above (16SuniversalFor and 16SuniversalRev) and generated a 462 bp product after 30 cycles of amplification at 95 °C for 1 min, 60 °C for 1 min and 72 °C for 1 min. PCR products were run on a 3% agarose gel containing ethidium bromide. The gel was visualized and quantitated using VisionWorks LS analysis software (Upland, CA) [66] . Accession codes: The metagenomic data have been deposited in the the BioProject database under accession code PRJNA231152 . How to cite this article: Ma, J. et al. High-fat maternal diet during pregnancy persistently alters the offspring microbiome in a primate model. Nat. Commun. 5:3889 doi: 10.1038/ncomms4889 (2014).